Dynamic and transformable Cu12cluster-based C-H···π-stacked porous supramolecular frameworks The assembly of cluster-based π-stacked porous supramolecular frameworks presents daunting challenges, including the design of suitable cluster building units, control of the sufficient C-H···π interactions, trade-off between structural dynamics and stability as well as understanding the resulting collective properties. Herein, we report a cluster-based C-H···π interaction-stacked porous supramolecular framework, namely, Cu12a-π, consisting of Cu 12 nanocluster as a 6-connected node, which is further propagated to a dynamic porous supramolecular frameworks via dense intralayer C-H···π interactions, yielding permanent porosity. In addition, Cu12a-π can be transformed into cluster-based nonporous adaptive crystals (Cu12b-NACs) via ligand-exchange following a dissociation-reassembly mechanism. Moreover, Cu12a-π can efficiently remove 97.2% of iodine from saturated iodine aqueous solutions with a high uptake capacity of 2.96 g·g −1 . These prospective results positioned at cluster-based porous supramolecular framework and enlighten follow-up researchers to design and synthesize such materials with better performance. Inspired by fascinating molecular pores that nature has evolved, scientists have made great progress in constructing porous materials [1] , [2] , [3] , [4] , [5] . Recently, a series of crystalline porous materials (CPMs) were assembled through intermolecular weak non-covalent interactions, which involve hydrogen bond [6] , [7] , [8] , [9] , [10] , π···π or C-H···π stacking [11] , [12] , [13] , [14] , [15] , [16] , electrostatic interactions, van der Waals forces [17] , [18] , etc. Wherein, π-stacked organic frameworks (πOFs), one of the newly emerging CPMs, have greatly broadened the boundaries of porous science, but few examples associated to such CPMs have been reported. Moreover, most of the reported πOFs are stabilized not merely by pure π···π stacking interactions, whereas other forces are also involved to a greater or lesser extent, e.g. C-H···π stacking interactions [12] . As a result, it is hard to figure out how much the C-H···π stacking interactions contribute the stability of CPMs. Therefore, the construction of supramolecular networks with permanent pores stabilized by C-H···π stacking interactions is meaningful to investigate the performance of such a non-covalent interaction in CPMs. In general, the CPMs stabilized by C-H···π interactions may show the similar dynamic behavior like third-generation MOFs due to the characteristic of non-covalent interactions, and can reversibly transform their structures in response to chemical guests via physical stimulation [19] , [20] , [21] . The rational construction of such CPMs may require the following two main factors: 1) the robust building unit; 2) the medium strength of the bridge linker, where the frame structure can balance the stability and flexibility. However, the most reported πOFs or HOFs (hydrogen-bonded organic frameworks) are constructed by organic building units, which may limit the stability on the process of dynamically structural transformation under drastic physical stimulation [22] , [23] . In addition, the further post-transformation of such OFs must be done through the redesign of the building unit. Therefore, the development of suitable building unit to rationally construct the C-H···π interaction-stacked porous supramolecular framework (PSF) with both dynamic structure and post-transformation is an important but currently challenging subject. To address these challenges, we designed a three-dimensional (3D) PSF, namely Cu12a-π , based on non-covalent C-H···π interactions between cluster-based building units that are protected by 9-(prop-2-yn-1-yl)−9H-carbazole (Cbz-PrAH) and p-tert -butylthiacalix[4]arene (H 4 TC4A). Of these, the Cbz-PrAH contains extended aromatic ring, which is conducive to the formation of intra- and intermolecular non-covalent C-H···π interactions [24] ; H 4 TC4A is a kind of macrocyclic ligand with intrinsic cavity structure [25] , [26] , [27] , [28] , [29] . As displayed in Fig. 1 , these features of two ligands synergistically lead to construct an as-prepared PSF ( Cu12a ), which can transform to guest-free PSF ( Cu12a-π ) through a dynamical single-crystal-to-single-crystal (SC-SC) fashion by removing guest molecules under heating and vacuum conditions. The monomer Cu 12 nanocluster as a zero-dimensional (0D) cluster-based building unit, can be further supramolecularly assembled into C-H···π interactions-stacked PSF. Even more impressively, the post-transformation of Cu12a-π followed a dissociation-reassembly mechanism, giving the cluster-based nonporous adaptive crystals (NACs) Cu12b-NACs with updates of both structure and properties. Fig. 1: Description of cluster-based PSF. Cartoon illustration showing the construction of cluster-based building unit. The Cu 12 cluster is further assembled into PSF via C-H···π interactions; NACs represent the nonporous adaptive crystals; the guest in Cu12a is ethyl acetate (EA) molecule. Full size image Synthesis and structural characterization To implement the synthesis of the as-prepared PSF, Cu12a , we selected copper(I) precursor, Cbz-PrACu (Please see experimental details in the Supplementary Methods) to react with H 4 TC4A via solvothermal method, giving the red rhombic crystals of Cu12a in a quite high yield of 91% (Supplementary Fig. 1 ). The process involved the depolymerization of the starting Cbz-PrACu precursor upon heating. Concomitantly, the H 4 TC4A was deprotonated, resulting in the formation of 12-nuclei copper(I) nanoclusters protected by Cbz-PrA ‒ and TC4A 4‒ ligands. The infrared (IR) spectroscopy confirmed the existence of Cbz-PrA ‒ in Cu12a. Besides, elements of Cu12a were confirmed by energy-dispersive x-ray (EDX) spectroscopy. More synthetic details and basic characterizations are listed in the Supplementary Figures and Tables (Supplementary Fig 2 – 4 and Supplementary Tables 1 , 2 ). 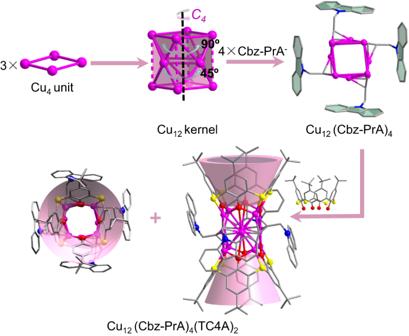Fig. 2: Structural anatomy of the Cu12cluster. Hydrogen atoms are removed for clarity. Color labels: purple, Cu; gray, C; red, O; blue, N; yellow, S. The pink cups represent the cavity structure of TC4A4‒. 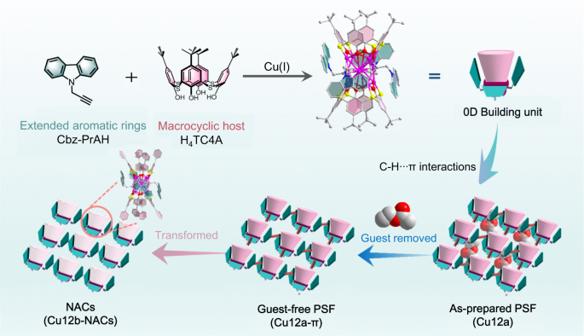Single-crystal X-ray diffraction (SCXRD) analyses revealed that the monomer of Cu12a crystallizes in a monoclinic unit cell under the P 2 1 / c space group with the asymmetric unit containing a half of nanocluster (Supplementary Fig. Fig. 1: Description of cluster-based PSF. Cartoon illustration showing the construction of cluster-based building unit. The Cu12cluster is further assembled into PSF via C-H···π interactions; NACs represent the nonporous adaptive crystals; the guest inCu12ais ethyl acetate (EA) molecule. 5 and Supplementary Table 1 ), and its formula is determined as [Cu 12 (Cbz-PrA) 4 (TC4A) 2 ]·(CH 3 COOCH 2 CH 3 ). The structural anatomy of the monomer was shown in Fig. 2 . The metal core can be viewed as an approximate cube-like pattern composed of three rectangular Cu 4 units rotated by 45° in sequence, the equatorial copper atoms are bulged from the centres of four vertical faces of the cube about 0.446 Å. The Cu 12 kernel exhibits a C 4 symmetry with a C 4 axis passing through the centres of two horizontal planes, and is consolidated by short Cu···Cu contacts (average distance of 2.76 Å), which are shorter than the sum of Bondi’s van der Waals radii of two Cu atoms (2.80 Å) [30] , implying an appreciable cuprophilic interactions. Furthermore, the types of capping ligands in the monomer of Cu12a are somewhat reminiscent of the Cu13a and Cu13b , where Cbz-PrA − and TC4A 4− capped on the periphery of the copper kernel in our previous work [31] . Fig. 2: Structural anatomy of the Cu 12 cluster. Hydrogen atoms are removed for clarity. Color labels: purple, Cu; gray, C; red, O; blue, N; yellow, S. The pink cups represent the cavity structure of TC4A 4‒ . Full size image The difference is that four Cbz-PrA − ligands like nails hold only one coordination mode (μ 4 -η 1 : η 1 : η 2 : η 2 , Supplementary Fig. 6a, b ), which are evenly distributed on the equator of the kernel, and their carbazole rings are oriented to two directions (up and bottom). The Cu-C bond lengths are in the range of 1.927 ~ 2.241 Å. Apart from the Cbz-PrA − ligands, the poles of the kernel are clutched by two TC4A 4− ligands. The phenolic hydroxyl and bridging sulfur donors of the TC4A 4− are bound to four copper atoms, showing the same coordination mode, μ 4 -κ o 2 :κ o 2 :κ o 2 :κ o 2 :κ s 1 :κ s 1 :κ s 1 :κ s 1 (Supplementary Fig. 6c ). The Cu-O and Cu-S bond lengths related to TC4A 4− fall in the ranges of 1.946 ~ 2.390 Å. The four Cbz-PrA − and two TC4A 4− ligands define the basic configuration of the Cu 12 cluster, and have substantial impacts on the crystal stability and adsorption behavior ( vide infra ). Crystalline supramolecular assembly Recently, the framework adaptability to guest uptake and stimuli-responsiveness are two intriguing features in flexible CPMs that are receiving increasing attentions [32] , [33] , [34] , [35] , [36] . Inspired by this, the guest EA molecules in Cu12a may endow it with similar behavior. Thus, the crystalline sample of Cu12a has been heated at 338 K upon vacuum for two days. Surprisingly, the activated sample of Cu12a , termed Cu12a-π , can still be analyzed via SCXRD, in which the guest EA molecules had been successfully removed to form permanent voids (Fig. 3a and Supplementary Fig. 7 ). Of note, heating under vacuum, the single crystal of Cu12a undergoes a phase transition at 338 K accompanied by a doubling of the crystallographic a axis and a change from the P 2 1 / c to C 2/ c space group. And the two-dimensional (2D) layers of Cu12a and Cu12a-π both adopt AA stacking mode, but the latter occurred with a distinct displacement between each layers along the ab plane, resulting in a slight reduction in the porosity (from 11.5% to 9.1%). Impressively, upon further soaking Cu12a-π in EA solvent for three days, the lattice again recovered to P 2 1 / c accompanied with the re-adsorption of the EA molecules. This indicates that the Cu12a and Cu12a-π as host matrixes can achieve reversible SC-SC transformation by removal and re-adsorption of the guest molecule, thus demonstrating the crystalline structural flexibility of Cu12a . Thermogravimetric analysis (TGA) (Fig. 3b ) indicates that the EA molecules in Cu12a are completely removed after phase transition and the Cu12a-π still remains stable even up to 558 K (Fig. 3b ). Besides that, the PXRD patterns of Cu12a and Cu12a-π exhibit distinct difference in peak positions and intensities, further verifying the occurrence of phase transition. Upon heating, the variable-temperature PXRD patterns of Cu12a-π show no change even up to 513 K, confirming its thermally robust structure (Fig. 3c ), which is superior than most reported πOFs [11] , [12] , [13] , [14] , [15] , [16] . Furthermore, after soaking Cu12a-π in different solvents (such as methanol: MeOH, acetonitrile: CH 3 CN, ethanol: EtOH, acetone: ACE, n-butanol: n BuOH and n-propanol: n PrOH) for at least 72 h at room temperature, their PXRD patterns were highly consistent well with the theoretical patterns of Cu12a , which demonstrated the framework highly dynamic stability to chemical solvents (Fig. 3d ). This excellence of thermal and chemical stabilities may be attributed to its unique molecular and packing structural features before and after phase transition. Fig. 3: The dynamics of PSF. a Reversible single-crystal-to-single-crystal transformation between Cu12a and Cu12a-π and corresponding unit cell parameters. b TGA and differential scanning calorimetry (DSC) curves of Cu12a and Cu12a-π . c Variable-temperature PXRD patterns of Cu12a-π . d PXRD patterns of Cu12a-π in different solvents. The guests in Cu12a are EA molecules. Full size image In Fig. 4a , trumpet-type Cu 12 cluster shows significant cavity structures above the poles of copper kernel, which is conductive to the close arrangement of cavity structures in one plane. And the higher rim of the cavity in Cu 12 cluster shows a maximum pore diameter of ~8.9 Å. Therefore, Cu 12 cluster can be regarded as a porous 0D cluster-based building unit, associated with two kinds of C-H···π interactions (C (sp3) -H···π (Cbz) =3.1 Å and C (sp2) -H···π (Cbz) =3.1 Å) between a carbazole ring and other carbazole ring, as well as between an allylene and a carbazole ring (Fig. 4b ), together supramolecular self-assembly into an extended PSF. As shown in Fig. 4c , the Cu 12 building units adopt 6-connected node to connect six adjacent building units to form a 2D ordered array, which undergoes obliquely slipped one-dimensional (1D) stacking via almost negligible interlayer H···H interactions (2.26 and 2.93 Å) of tertiary butyl to form a final 3D supramolecular framework (Fig. 4d ). Of these, the intralayer C-H···π interactions contribute to the framework stability as the dominant linkages compared to the strength of weak interlayer H···H interactions [37] . By contrast, the supramolecular crystalline assembly of Cu 12 cluster in Cu12a also exhibits a similar mode to Cu12a-π (Supplementary Fig. 8 ), except for the relative large diameter of pore ( ~ 9.3 Å) and length of intralayer bridges (C (sp3) -H···π (Cbz) =3.2 or 3.4 Å and C (sp2) -H···π (Cbz) =2.8 Å) due to the incorporation of guest EA solvents. Fig. 4: Supramolecular assembly of PSF. a The Cu 12 cluster in Cu12a-π displays a trumpet-type motif. b The intralayer C-H···π interactions between Cu 12 clusters. The top ( c) and side ( d) views of local PSF. e Left: N 2 adsorption and desorption isotherms of Cu12a-π at 77 K; f The CH 4 , CO 2 , C 2 H 4 and C 2 H 6 adsorption-desorption isotherms of Cu12a-π at 273 (Left) and 293 K (Right). The sample weight of Cu12a-π in gas sorption measurements: 100 mg. Full size image On the basis of packing characteristic of Cu12a-π , it is clearly seen that the small cavities provided by the thiacalix[4]arene and permanent voids between each layers effectively endow the Cu12a-π with certain porosity (Supplementary Fig. 7 ). Correspondingly, analysis of N 2 adsorption isotherms of Cu12a-π gives rise to a Brunauer-Emmett-Teller (Langmuir) surface area of 31.93 (45.29) m 2 ·g −1 , and a wide pore size distribution in the range of 0.8–1.6 nm calculated by Horvath-Kawazoe (HK) model (Fig. 4e and Supplementary Fig. 9 ). These results are thought to reflect the small cavities provided by the thiacalix[4]arene and the voids between the 2D layers. Meanwhile, Fig. 4f shows the pure-component equilibrium adsorption isotherms for the CH 4 , CO 2 , C 2 H 4 , and C 2 H 6 collected at different temperatures. The maximum C 2 H 6 uptake reaches 30.48 cm 3 ·g −1 (273 K) at normal pressure, further confirming the real existence of permanent porosity in Cu12a-π . Transformed into NACs Remarkably, post-modification has been one of the research hotspots for MOFs in recent years, facilitating the acquisition of anticipant structures and properties [38] , [39] , [40] , [41] . Inspired by this, the Cu 12 nanocluster acting as a building unit may feature ligand-exchange to remodel the PSFs. Therefore, we tried to transform Cu12a-π by dissolving crystalline samples in an isopropanol/tetrahydrofuran (v:v = 3:3) mixture, to which an excess of H 4 PTC4A ( p-phenyl -thiacalix[4]arene) was added, and then the above solution continued to react under solvothermal condition to generate red block crystals of Cu12b . Except for the p-phenyl -thiacalix[4]arene (Supplementary Fig. 5d ), the monomer Cu 12 cluster in Cu12b has similar compositions to that of Cu12a , and the four phenyl groups act as the up rim of cavity structure (Fig. 5a ). In view of the significantly different optical absorbance between the two Cu 12 clusters (Supplementary Fig. 10a ), we carried out the time-course optical absorptions to monitor the conversion process (Fig. 5b ). With time going on, the intensity of its characteristic absorption peak at ~300 nm increased significantly upon stirring, as well as the peak at ~340 nm gradually changed from a prominent peak to a shoulder peak. Meanwhile, the color of the mixture solution transformed from yellow to pale yellow and finally to brownish yellow (Supplementary Fig. 10b ). So as to intuitively visualize the trend of the two characteristic peaks, the correlation between the absorbance ratio of the two peaks and reaction time was illustrated. As the time went from 0 to 105 min, the value of A 300 nm /A 340 nm was raised from 1.563 to a maximum of 2.361, and then maintained around 2.335 for Cu12b (Supplementary Fig. 10c ). Considering the following factors: (i) the extra charge transition of IL (Cbz-PrA+PTC4A) CT in Cu12b leading to the variation in the absorption intensity of the two nanoclusters at ~300 nm (Please see details in the Supplementary Methods); (ii) the position of the maximum absorption peaks of the two ligands (H 4 TC4A and H 4 PTC4A) (Supplementary Fig. 10d ); (iii) dynamic characteristics of coordination bonds, we tentatively concluded that the increase of absorption strength in A 300 nm /A 340 nm may be attributed to the dissociation of TC4A 4‒ and bonding of PTC4A 4‒ ligands in Cu12a , leading to the increase in the absorption intensity of whole system near 300 nm. When the dissociation and bonding were in equilibrium, the A 300 nm /A 340 nm reached its crest values. Fig. 5: The transformation of PSF. a Structural transformation of monomer Cu 12 cluster from Cu12a to Cu12b . b UV‒Vis absorption spectra of the conversion from Cu12a to Cu12b over the time course at 293 K. c, d Positive-ion mode ESI-MS of the crystals of Cu12a ( a ) and Cu12b ( d ) dissolved in mixed CHCl 3 and CH 3 OH. Inset: The zoom-in mass spectrum of experimental (green line) and simulated (red line) isotope-distribution patterns of each labeled species. e Time-course ESI-MS of transformation from Cu12a to Cu12b induced by adding H 4 PTC4A. Full size image To verify the assumption on the transformation mechanism, we monitored the ligand-exchange process in the structural transformation from Cu12a to Cu12b by electrospray ionization mass spectrometry (ESI-MS). As shown in Fig. 5c, d , the Cu12a and Cu12b in mixed CH 3 OH and CHCl 3 exhibit a series of +1 species ( 1a - 1e for Cu12a ; 2a-2i for Cu12b ) at the m/z range of 3010-3090 and 3170-3345, respectively, which correspond to their intact cluster bound with different cations or solvents. The most dominant peak 1b at m/z 3036.9040 and peak 2b at m/z 3196.6478 can be attributed to [Cu 12 (TC4A) 2 (Cbz-PrA) 4 Na] + (Cal. 3036.8907) and [Cu 12 (PTC4A) 2 (Cbz-PrA) 4 Na] + (Cal. 3196.6410), respectively. However, as the reaction of H 4 PTC4A and Cu12a proceeded in CHCl 3 , the parent peaks of Cu12a ( 1a − 1e ) progressively faded away within 20 min (Fig. 5e ), which involves the dissociation of the cluster. Of note, an intermediate species ( 3a ) appeared at 30 min, and can be assigned to [Cu 12 (PTC4A)(TC4A)(Cbz-PrA) 4 H] + . This species 3a is the mono-substituted product of Cu12a , in which one of the TC4A 4- ligands is replaced by PTC4A 4- . After 80 min, we observed a species 2j , [Cu 12 (PTC4A) 2 (Cbz-PrA) 4 (CH 3 OH)(H 2 O) 2 K] + , which can be identified as the bis-substituted product of Cu12a . This result indicates that Cu12b is more thermodynamically stable than Cu12a , which also was confirmed by DFT calculations (Supplementary Fig. 11 ). Moreover, the collision-induced dissociation (CID) mass further demonstrated the higher stability of Cu12b than Cu12a in gas phase (Please see details in the Supplementary Figures). 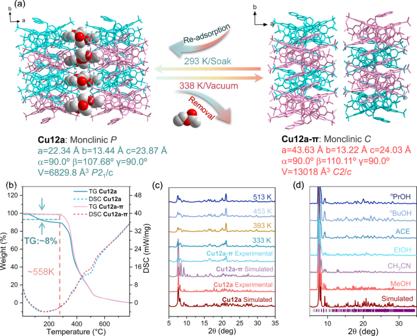Fig. 3: The dynamics of PSF. aReversible single-crystal-to-single-crystal transformation betweenCu12aandCu12a-πand corresponding unit cell parameters.bTGA and differential scanning calorimetry (DSC) curves ofCu12aandCu12a-π.cVariable-temperature PXRD patterns ofCu12a-π.dPXRD patterns ofCu12a-πin different solvents. The guests inCu12aare EA molecules. More formula assignments for the above species in ESI-MS were performed as listed in Supplementary Table 3 . The transformation between the two Cu 12 clusters was initially presumed to be a simple ligand-exchange process based on the single crystal structure and optical monitoring. However, further investigation using ESI-MS tracking revealed that this transformation was not a straightforward ligand-substitution, but rather a kinetically driven dissociation of the initial cluster, followed by a reassembly to form a thermodynamically stable new cluster. Thus, we have established the dissociation-reassembly (DR) mechanism to describe above transformation process, highlighting the dynamic nature of the dissociation and subsequent reassembly steps. The DR mechanism provides a conceptual framework to understand the intricate dynamics involved in the transformation of Cu12a to the more stable Cu12b [42] , [43] , [44] , [45] , [46] , [47] , [48] , [49] , [50] . Considering the deep cavity of PTC4A 4‒ , we further checked the packing formed by Cu 12 cluster in Cu12b . There is one THF molecule residing in the cavity of each PTC4A 4‒ in Cu12b , which reduces the void produced by PTC4A 4‒ ligand itself, so the Cu12b is a nonporous structure. The activated experiment of Cu12b was further carried out, and the activated sample namely Cu12b-NACs had been successfully removed the guest THF solvents (Supplementary Fig. 12 ). Of note, Cu12b-NACs also undergoes a SC-SC phase transition accompanied by a trebling of the crystallographic volume. Due to the removal of THF molecules in both lattice and the cavity of PTC4A 4‒ , the Cu 12 clusters are shifted to more closer, producing deeper interpenetration between the upper phenyl rings of adjacent PTC4A 4‒ compared to those in Cu12b , where the THF molecules block interpenetration (Supplementary Fig. 13 ). Thus, the Cu12b-NACs can be viewed as cluster-based nonporous adaptive crystals (NACs), which are relatively nonporous but with medium surface areas [51] , [52] , [53] , [54] , [55] , [56] . In light of this, the analysis of N 2 adsorption isotherm of Cu12b-NACs gives an experimental Brunauer-Emmett-Teller (Langmuir) surface area of 14.88 (12.63) m 2 ·g -1 , which is less than half of that of Cu12a-π , and the pore-size distribution exhibits broad and ambiguous peak (Supplementary Fig. 14 ), which further verifies that Cu12b-NACs acting as the NAC features medium surface area and non-porosity. We also performed the gas adsorption experiments of Cu12b-NACs at 273 K, and the uptake amounts of CH 4 , CO 2 , C 2 H 4 and C 2 H 6 decreased a half compared to that of Cu12a-π . This observation fits the fact of condensed stacking of crystallographic structure. Iodine adsorption It is well known that capturing iodine with high adsorption capacity from aqueous solution remains a challenge for most porous materials [57] , [58] , [59] , [60] , [61] , [62] , [63] , [64] . Benefiting from the permanent porosity of Cu12a-π and the potentially adaptive absorption capacity of Cu12b-NACs , the capacities of iodine uptake would be worthy of further investigation, especially in aqueous solution. Hence, adsorption experiments involved with saturated aqueous solutions of iodine were performed. In this case, the UV‒Vis spectra of this aqueous solutions show a weakening of the absorption profile with time in the presence of Cu12a-π and Cu12b-NACs (Fig. 6a, b and Supplementary Fig. 15 – 17 ). The Cu12a-π needs much more time to reach equilibrium, but shows higher uptake efficiency compared to Cu12b-NACs . 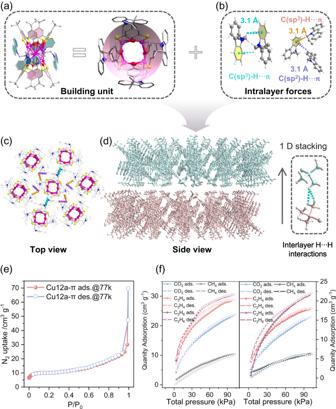Fig. 4: Supramolecular assembly of PSF. aThe Cu12cluster inCu12a-πdisplays a trumpet-type motif.bThe intralayer C-H···π interactions between Cu12clusters. The top (c)and side (d)views of local PSF.eLeft: N2adsorption and desorption isotherms ofCu12a-πat 77 K;fThe CH4, CO2, C2H4and C2H6adsorption-desorption isotherms ofCu12a-πat 273 (Left) and 293 K (Right). The sample weight ofCu12a-πin gas sorption measurements: 100 mg. Wherein, Cu12a-π shows an iodine adsorption efficiency of 97.2% from aqueous solution within 60 min, with a total iodine uptake of 2.96 g·g ‒1 , which was superior to most reported iodine adsorbents (Supplementary Table 4 ). Although, because of the relatively nonporous feature caused by the offset of p-phenyl -thiacalix[4]arene on the packing of Cu12b-NACs , the uptake efficiency of iodine was about 89.42%, with an equilibrium uptake of 2.73 g·g ‒1 . Therefore, we can draw a preliminary conclusion that the iodine adsorption sites of the Cu12a-π and Cu12b-NACs are not only the cavity of the supramolecular framework, but also are related to the surface areas of crystal. The scanning electron microscopy (SEM) image of I 2 @Cu12a-π showed the crystal-like morphology (Fig. 6c ), and the PXRD pattern of Cu12a-π soaked in aqueous solution shows similar diffraction peaks to Cu12a-π , indicating its excellent framework stability. Of note, I 2 @Cu12a-π still shows obvious diffraction peaks, suggesting that the framework of Cu12a-π was not interrupted after iodine adsorption (Fig. 6d ). Besides, the Cu12a-π also shows some degree of recyclable ability and can be further reused for additional iodine adsorption tests via soaking I 2 @Cu12a-π in EA solvent (Supplementary Fig. 18 ). Fig. 6: Iodine adsorption of PSF. a Time-dependent adsorption profiles for the Cu12a-π and Cu12b-NACs (0.1 mg·mL ‒1 ) when immersed in 30 mL iodine aqueous solutions (1.2 mM). b UV‒Vis spectra of saturated iodine aqueous solutions before and after adsorption by Cu12a-π and Cu12b-NACs , respectively; the inset shows the color changes of the iodine aqueous solution after adsorption by Cu12a-π and Cu12b-NACs , respectively. c SEM and EDX images of I 2 @Cu12a-π , scan bar = 100 μm. d PXRD patterns of Cu12a-π, Cu12a-π in H 2 O and I 2 @Cu12a-π . e UV‒Vis spectra of Cu12a-π, I 2 @Cu12a-π and I 2 . The inset shows color change of the Cu12a-π before (left) and after (right) adsorbing iodine. f XPS spectrum of I 2 @Cu12a-π . Full size image Due to its relatively high iodine adsorption capacity, Cu12a-π was chosen as the ideal sample to verify that the iodine was present as polyiodide ions after adsorption. For this, the UV‒Vis absorption, energy-dispersive x-ray spectroscopy were carried out. The UV‒Vis absorption spectra of Cu12a-π and the pristine iodine showcase a significantly different absorption profile compared to I 2 @Cu12a-π (Fig. 6e ) in the solid state. Both the Cu12a-π and pristine iodine exhibit weak absorption intensity beyond 900 nm, yet the latter exhibits a broad tail peak over the 1000 nm. The strong absorption of I 2 @Cu12a-π in near-infrared region may be attributed to the charge transfer between polyiodide anions (mainly I 3 − and I 5 − ) and Cu12a-π , which has been reported previously for iodine adsorption materials [65] , [66] . Moreover, the I 3d X-ray photoelectron spectrum (XPS) of I 2 @Cu12a-π was measured, and two broad peaks at ~620 and ~632 eV indicate the presence of the I 3 ‒ and I 5 ‒ anions, respectively (Fig. 6f ). In summary, we have successfully developed a dynamic and transformable 3D PSF ( Cu12a-π ) with cluster-based building units held together through intralayer non-covalent C-H··π interactions. The Cu12a-π is successfully constructed through the SC-SC transformation by the removal of guest molecules from pristine Cu12a , showing unexpected structural dynamics and superior thermal stability than most reported π-stacked frameworks. 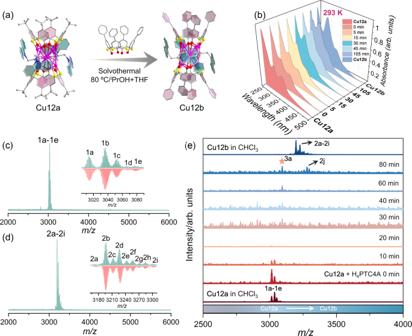Fig. 5: The transformation of PSF. aStructural transformation of monomer Cu12cluster fromCu12atoCu12b.bUV‒Vis absorption spectra of the conversion fromCu12atoCu12bover the time course at 293 K.c,dPositive-ion mode ESI-MS of the crystals ofCu12a(a) andCu12b(d) dissolved in mixed CHCl3and CH3OH. Inset: The zoom-in mass spectrum of experimental (green line) and simulated (red line) isotope-distribution patterns of each labeled species.eTime-course ESI-MS of transformation fromCu12atoCu12binduced by adding H4PTC4A. 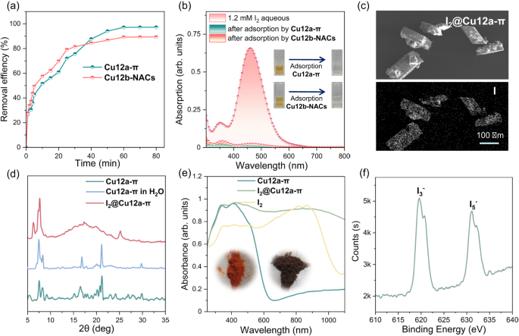Fig. 6: Iodine adsorption of PSF. aTime-dependent adsorption profiles for theCu12a-πandCu12b-NACs(0.1 mg·mL‒1) when immersed in 30 mL iodine aqueous solutions (1.2 mM).bUV‒Vis spectra of saturated iodine aqueous solutions before and after adsorption byCu12a-πandCu12b-NACs, respectively; the inset shows the color changes of the iodine aqueous solution after adsorption byCu12a-πandCu12b-NACs, respectively.cSEM and EDX images ofI2@Cu12a-π, scan bar = 100 μm.dPXRD patterns ofCu12a-π,Cu12a-π in H2OandI2@Cu12a-π.eUV‒Vis spectra ofCu12a-π,I2@Cu12a-πandI2. The inset shows color change of theCu12a-πbefore (left) and after (right) adsorbing iodine.fXPS spectrum ofI2@Cu12a-π. Moreover, the changing in upper rim of thiacalix[4]arene, Cu12a-π can be transformed into the nonporous adaptive crystal Cu12b-NACs following a DR mechanism, realizing the structural and performance updates. Based on the permanent porosity, Cu12a-π can absorb iodine in aqueous solution reaching a high capacity of 2.96 g·g ‒1 . Overall, all unique structural features as well as the iodine adsorption performance of such cluster-based PSF are indicative of a bright future of this type of porous materials. Syntheses of the As-prepared PSFs Cu12a Cbz-PrACu (5.00 mg, 0.02 mmol) and H 4 TC4A (13.0 mg, 0.02 mmol) were mixed in 6.00 mL methanol/ethyl acetate (v:v = 3:3). The resulting suspension was sealed and heated at 80 °C for 2000 min. After cooling to room temperature, red crystals of Cu12a were formed (4.57 mg; yield: 91%). Selected IR peaks (cm −1 ): 2950 (s), 2906 (w), 2860 (w), 1732 (s), 1584 (m), 1450 (s), 1364 (m), 1315 (m), 1257 (s), 1208 (m), 1037 (m), 926 (w), 885 (w), 840 (s), 751 (s), 711 (s), 625 (w), 531 (m). Cu12b The crystals of Cu12a (4.57 mg, 1.52 μmol) were dissolved in mixed solvents of 6.00 mL isopropanol/tetrahydrofuran (v:v = 3:3), then H 4 PTC4A (16.0 mg, 0.02 mmol) was added successively. The resulting suspension was sealed and heated at 80 °C for 2000 min. After cooling to room temperature, red crystals of Cu12b were formed (2.07 mg; yield: 43%). Selected IR peaks (cm −1 ): 2955 (s), 2901 (w), 2865 (w), 1777 (w), 1589 (m), 1454 (s), 1364 (m), 1311 (s), 1255 (s), 1202 (m), 916 (w), 876 (w), 831 (s), 741 (s), 714 (s), 616 (w), 526 (m).